The genome of a Mesozoic paleovirus reveals the evolution of hepatitis B viruses Paleovirology involves the identification of ancient endogenous viral elements within eukaryotic genomes. The evolutionary origins of the reverse-transcribing hepatitis B viruses, however, remain elusive, due to the small number of endogenized sequences present in host genomes. Here we report a comprehensively dated genomic record of hepatitis B virus endogenizations that spans bird evolution from >82 to <12.1 million years ago. The oldest virus relic extends over a 99% complete hepatitis B virus genome sequence and constitutes the first discovery of a Mesozoic paleovirus genome. We show that Hepadnaviridae are >63 million years older than previously known and provide direct evidence for coexistence of hepatitis B viruses and birds during the Mesozoic and Cenozoic Eras. Finally, phylogenetic analyses and distribution of hepatitis B virus relics suggest that birds potentially are the ancestral hosts of Hepadnaviridae and mammalian hepatitis B viruses probably emerged after a bird–mammal host switch. Our study reveals previously undiscovered and multi-faceted insights into prehistoric hepatitis B virus evolution and provides valuable resources for future studies, such as in-vitro resurrection of Mesozoic hepadnaviruses. The emerging field of paleovirology [1] has discovered a wealth of endogenous viral elements (EVEs) [2] scattered within eukaryotic genomes. Surprisingly, in addition to the retroviral origin of many EVEs, all other major groups of eukaryotic viruses exhibit a more or less pronounced genomic record of endogenizations, too [3] . Such genomic relics arise as a consequence of viral infiltration of the host’s germline, followed by insertion and fixation of virus-derived DNA fragments within the host’s genome [4] , [5] . As each virus relic is present at a specific genomic location, the presence/absence patterns of orthologous EVE insertions among closely and less closely related species permit the reconstruction of the lower and upper age boundary of endogenization events [3] . Hepatitis B viruses (HBVs) belong to the Hepadnaviridae family of reverse-transcribing DNA viruses and constitute a major global health issue by infecting more than a third of the human population [6] . Until very recently [2] , [7] , these viruses were presumed to completely lack a record of genomic endogenizations, as none of the sequenced genomes of their extant avian, rodent and primate hosts [8] (that is, human, chimp, gorilla, orangutan, gibbon) exhibit HBV-derived sequences. Consequently, insights into the evolutionary origin of Hepadnaviridae were based solely on sequence analyses of extant HBVs, dating the last common ancestor of Orthohepadnaviridae and Avihepadnaviridae to 30,000 years [9] or 125,000 years [10] ago. It was rather the recently published [11] genome of the zebra finch, a bird species that is not documented to be an extant HBV host [8] , that revealed the first evidence for HBV-derived EVEs in BLAST [12] -based analyses [2] , [7] . Gilbert and Feschotte [7] identified about a dozen HBV-derived fragments, each with a length extending over ~4 to ~40% of the extant duck HBV (DHBV) genome, and revealed compelling evidence that at least one of these EVEs was inserted as early as >19 million years ago (MYA). Here, we report a dated record of HBV germline infiltrations in the lineage leading to the zebra finch that discloses even more far-reaching surprises. We conducted comprehensive presence/absence analyses ( Supplementary Table S1 ) of previously [2] , [7] and newly detected HBV-derived EVEs in the zebra finch genome ( Supplementary Table S2 ) using a dense taxon sampling, permitting the reconstruction of HBV endogenization events during bird evolution and revealing the 99% complete genome sequence of a paleovirus nested within an intron of the FRY (that is, Drosophila Furry homolog) gene. Hepadnavirus endogenizations and bird evolution From the 12 endogenous zebra finch HBV-derived EVEs (eZHBVs) recognizable via tBLASTx (see Methods), we were able to amplify eight insertion loci in all those bird species that are necessary for a precise reconstruction of the respective insertion event. The resultant eZHBV presence/absence patterns ( Supplementary Table S1 ) revealed HBV endogenizations during bird evolution in different geological epochs ( Fig. 1 ). The youngest HBV-derived EVE (eZHBV_M) is present in the zebra finch and absent in the orthologous position in all other sampled taxa; thus, its insertion occurred <12.1 MYA during the Miocene or even more recently. Six of our eight dated EVEs are either of Oligocene (eZHBV_O1-O5; 26.6-34.2 MYA) or Eocene (eZHBV_E; 34.2-35 MYA) origin, as they are present in passeroid songbirds to the exclusion of either leafbirds and sunbirds or sunbirds alone. Strikingly, we identified an even older eZHBV insertion (eZHBV_C) that is shared among all major neoavian clades sensu [13] and absent in non-neoavian taxa (for example, chicken), strongly suggesting that this HBV endogenization occurred in the common ancestor of Neoaves. As both the most conservative [14] and the most comprehensive [15] molecular analyses date the existence of the neoavian ancestor to >74 MYA [14] or 82–94 MYA [15] , the neoavian-wide presence ( Fig. 2 ) of eZHBV_C provides direct evidence for the existence and endogenization of Hepadnaviridae during the Upper Cretaceous. The hepadnaviral genomic record of germline infiltrations is thus considerably older than previously assumed [7] . Even more surprisingly, the eZHBV_C EVE constitutes a continuous and 99% complete paleovirus genome sequence ( Fig. 3a ) that has been buried in neoavian genomes since the Mesozoic Era. 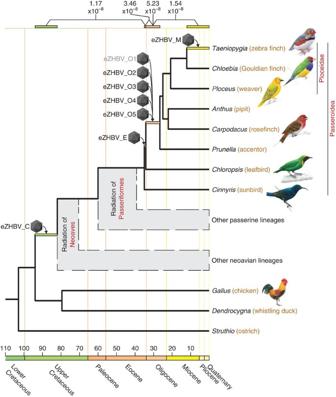Figure 1: Hepatitis B virus endogenization events during bird evolution. Presence/absence analyses of zebra finch HBV EVE insertion loci (Supplementary Table S1; for full alignments, seeSupplementary Data 1) revealed eZHBV endogenization events in the ancestor of Neoaves, during early passeroid evolution and during recent ploceid evolution. The avian tree of life13,34is shown as a simplified chronogram based on molecular dates of interordinal avian relationships15, as well as relationships within Passeriformes32and Ploceidae (Supplementary Fig. S1). Based on HASs of the dated EVEs, nucleotide substitution rates (in substitutions/site/year) were calculated (Supplementary Table S3) for the respective parts of eZHBV evolution and denoted above the tree. Endogenization events are depicted as icosahedrons and temporal ranges of insertion events are shown as coloured rectangles (colours correspond to the respective geological epoch in the International Stratigraphic Chart;http://www.stratigraphy.org/ics%20chart/09_2010/StratChart2010.pdf). Although eZHBV_O1 (grey letters) was previously dated7, we sampled two missing taxa (Prunella,Chloropsis) that permit a more precise dating. Figure 1: Hepatitis B virus endogenization events during bird evolution. Presence/absence analyses of zebra finch HBV EVE insertion loci ( Supplementary Table S1 ; for full alignments, see Supplementary Data 1 ) revealed eZHBV endogenization events in the ancestor of Neoaves, during early passeroid evolution and during recent ploceid evolution. The avian tree of life [13] , [34] is shown as a simplified chronogram based on molecular dates of interordinal avian relationships [15] , as well as relationships within Passeriformes [32] and Ploceidae ( Supplementary Fig. S1 ). Based on HASs of the dated EVEs, nucleotide substitution rates (in substitutions/site/year) were calculated ( Supplementary Table S3 ) for the respective parts of eZHBV evolution and denoted above the tree. Endogenization events are depicted as icosahedrons and temporal ranges of insertion events are shown as coloured rectangles (colours correspond to the respective geological epoch in the International Stratigraphic Chart; http://www.stratigraphy.org/ics%20chart/09_2010/StratChart2010.pdf) . Although eZHBV_O1 (grey letters) was previously dated [7] , we sampled two missing taxa ( Prunella , Chloropsis ) that permit a more precise dating. 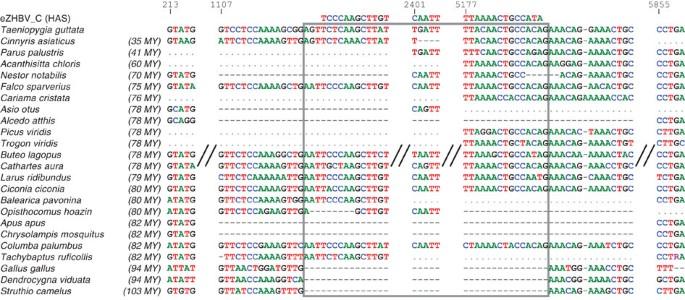Figure 2: Presence/absence pattern of the Mesozoic eZHBV_C paleovirus within avian genomes. Non-neoavian representatives (Gallus,Dendrocygna,Struthio) exhibit the ancestral absence situation, whereas neoavian representatives exhibit the unambiguous presence of the eZHBV_C fragment. InAlcedo,ApusandChrysolampis, birds that are each phylogenetically nested34within Neoaves, large and unspecific deletions have led to the secondary loss of almost the complete intron (spanning the paleovirus + flanking sequences). Approximate dates of species divergence15,32to the zebra finch (Taeniopygia) are shown in italicized letters. The eZHBV_C presence/absence region is boxed and aligned to the HAS of eZHBV_C. Missing sequence information is denoted as grey dots and numbers denote positions in the full alignment of the eZHBV_C locus (Supplementary Data 1). Full size image Figure 2: Presence/absence pattern of the Mesozoic eZHBV_C paleovirus within avian genomes. Non-neoavian representatives ( Gallus , Dendrocygna , Struthio ) exhibit the ancestral absence situation, whereas neoavian representatives exhibit the unambiguous presence of the eZHBV_C fragment. In Alcedo , Apus and Chrysolampis , birds that are each phylogenetically nested [34] within Neoaves, large and unspecific deletions have led to the secondary loss of almost the complete intron (spanning the paleovirus + flanking sequences). Approximate dates of species divergence [15] , [32] to the zebra finch ( Taeniopygia ) are shown in italicized letters. The eZHBV_C presence/absence region is boxed and aligned to the HAS of eZHBV_C. Missing sequence information is denoted as grey dots and numbers denote positions in the full alignment of the eZHBV_C locus ( Supplementary Data 1 ). 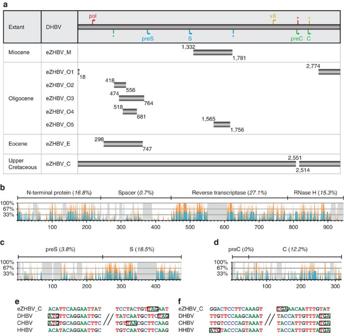Figure 3: Genome organisation and sequence conservation of the Mesozoic hepatitis B paleovirus (eZHBV_C). (a) The HAS of the eZHBV_C insertion covers ~99% of the circular 3,024-bp extant DHBV genome (AY494851), whereas the other seven dated EVEs are HBV genome fragments that range from 4.6% (eZHBV_O2) to 14.7% (eZHBV_E and eZHBV_M) coverage. For the DHBV genome, the start (arrow) and stop (asterisk) codon positions for the ORFs of the polymerase protein22(pol; red), the presurface/surface protein22(preS/S; blue), and the precore/core protein22(preC/C; green) are shown, as well as the putative location of the structural vestige of an X protein21(vX; orange). (b–d) The pol (b), preS/S (c) and preC/C (d) proteins of the eZHBV_C HAS exhibit amino-acid positions (for full alignments, seeSupplementary Data 2) that are both conserved among extant avian HBVs (blue graph) and among extant mammalian HBVs (orange graph). The proportions of perfectly conserved sites (that is, 100% conservation) within the respective regions of each ORF are denoted as italicized percentages and alignment gaps in the eZHBV_C sequence are shown as grey background. (e,f) The eZHBV_C HAS lacks an intact start codon for the structural prediction of a vestigial X protein21(e) of DHBV and crane HBV (CHBV), as well as an intact ORF for the X-like protein22(f) of heron HBV (HHBV). Intact start (ATG) and stop (TAA/TGA) codons are boxed. Full size image Figure 3: Genome organisation and sequence conservation of the Mesozoic hepatitis B paleovirus (eZHBV_C). ( a ) The HAS of the eZHBV_C insertion covers ~99% of the circular 3,024-bp extant DHBV genome (AY494851), whereas the other seven dated EVEs are HBV genome fragments that range from 4.6% (eZHBV_O2) to 14.7% (eZHBV_E and eZHBV_M) coverage. For the DHBV genome, the start (arrow) and stop (asterisk) codon positions for the ORFs of the polymerase protein [22] (pol; red), the presurface/surface protein [22] (preS/S; blue), and the precore/core protein [22] (preC/C; green) are shown, as well as the putative location of the structural vestige of an X protein [21] (vX; orange). ( b – d ) The pol ( b ), preS/S ( c ) and preC/C ( d ) proteins of the eZHBV_C HAS exhibit amino-acid positions (for full alignments, see Supplementary Data 2 ) that are both conserved among extant avian HBVs (blue graph) and among extant mammalian HBVs (orange graph). The proportions of perfectly conserved sites (that is, 100% conservation) within the respective regions of each ORF are denoted as italicized percentages and alignment gaps in the eZHBV_C sequence are shown as grey background. ( e , f ) The eZHBV_C HAS lacks an intact start codon for the structural prediction of a vestigial X protein [21] ( e ) of DHBV and crane HBV (CHBV), as well as an intact ORF for the X-like protein [22] ( f ) of heron HBV (HHBV). Intact start (ATG) and stop (TAA/TGA) codons are boxed. Full size image Long-term substitution rates of Hepadnaviridae On the basis of the orthologous eZHBV sequences obtained in our presence/absence screenings of each of the eight EVEs, we derived (see Methods) hypothetical ancestral sequences (HASs) for further sequence analyses, as we expect that these HASs approximate the respective sequence condition of each HBV fragment at the time of its endogenization. By combining pairwise HAS divergences ( Supplementary Table S3 ) with the dating of the upper and lower boundaries of each HBV endogenization event, we calculated long-term nucleotide substitution rates ( Supplementary Table S3 ) during the different prehistoric chapters of HBV evolution ( Fig. 1 ). Notably, the lowest substitution rates are found when comparing Mesozoic versus Eocene eZHBVs (that is, 1.17 × 10 −8 substitutions per site per year) as well as Oligocene versus Miocene eZHBVs (that is, 1.54 × 10 −8 substitutions per site per year), whereas Eocene versus Oligocene and Oligocene versus Oligocene eZHBV comparisons resulted in slightly higher values (3.46 × 10 −8 and 5.23 × 10 −8 substitutions per site per year). All these eZHBV substitution rates are similar to previous estimations [7] (based on pairwise comparisons of eZHBVs versus extant avian HBVs) and suggest that the Mesozoic and Cenozoic long-term substitution rates of Hepadnaviridae are more than 1,000-fold slower [7] than the extant short-term substitution rates of human HBVs [16] , even during their e-antigen positive phase [17] . Genome evolution of Hepadnaviridae Our study provides direct evidence that the compact genomic organisation of Hepadnaviridae has remained largely unchanged for the last >82 MYA of hepadnaviral evolution. This assumption is based on the presence of partially overlapping polymerase (pol), presurface/surface (preS/S) and precore/core (preC/C) open reading frames (ORFs) [8] in the HAS of the 99% complete Mesozoic paleovirus genome (eZHBV_C). Furthermore, our analyses of extant HBV and paleoviral eZHBV_C protein sequences unravel an unexpected degree of amino-acid sequence conservation in certain regions of HBV genomes ( Fig. 3b–d ). Most strikingly, the reverse transcriptase region of the pol ORF exhibits 27.1% perfectly conserved amino-acid positions ( Fig. 3b ), but also other genomic regions (for example, N-terminal protein, RNase H, S ORF, C ORF) are thoroughly conserved at 12.2–18.5% of their amino-acid sites ( Fig. 3b–d ). Merely the spacer region of the pol ORF, the preC-specific region, and the preS-specific region show a relatively low proportion (that is, <5%) of unvaried amino-acid positions ( Fig. 3b–d ). Despite their genomic similarities, the most striking difference between Orthohepadnaviridae and Avihepadnaviridae is the presence of an X protein in the genomes of human and other mammalian HBVs [8] , a regulatory protein with multiple protein-interacting functions [18] , [19] , [20] and a tumor-promoting effect [18] . When we thus performed tBLASTn searches of mammalian HBV X proteins in the eZHBV_C genome, we found no evidence for the presence of an intact or at least a degenerated X ORF in this Mesozoic paleovirus. Additionally, nucleotide sequence alignments of eZHBV_C and extant avian HBVs revealed that eZHBV_C lacks the hypothetical start codon of an X-like ORF that has been annotated in some Avihepadnaviridae based on the structural prediction sensu [21] ( Fig. 3e ) or the ORF prediction sensu [22] ( Fig. 3f ). Thus, our paleovirological indication for the absence of the X ORF in a Mesozoic paleovirus suggests that, in contrast to previous assumptions [10] , [21] , the oncogenic X protein of Orthohepadnaviridae might not have been present in the common ancestor of Hepadnaviridae. Instead, it probably emerged de novo via overprinting [23] of pol and precore ORF parts in the common ancestor of mammalian HBVs. Phylogeny of Hepadnaviridae Our phylogenetic analyses of the pol protein from eZHBV HASs and extant HBVs reveal three ancient lineages of zebra finch eZHBV EVEs (also when including very recently published [24] , [25] budgerigar HBV EVEs, Supplementary Fig. S3 ) and further insights into early hepadnaviral evolution ( Fig. 4 ). The Eocene/Oligocene EVEs (eZHBV_E +eZHBV_O1-O5) group as sister to extant avian HBVs, whereas the youngest (eZHBV_M) and the oldest (eZHBV_C) HBV-derived EVEs each appear to be independent lineages that are rather distantly related to extant avian HBVs. The exact branching order of eZHBV_M and eZHBV_C in relation to extant HBVs depends on the position of the root in the HBV phylogeny. When the tree is rooted to mammalian HBVs ( Fig. 4a ), the EVE record and tree topology imply that Orthohepadnaviridae and Avihepadnaviridae separated before the endogenization of eZHBV_C, that is, >94 to >82 MYA. Accordingly, the ancestor of Hepadnaviridae probably infected the amniote ancestor that lived >324 MYA [26] and subsequently diverged into avian and mammalian HBVs with the emergence of the bird and mammal lineages, respectively. As an alternative to this codivergence scenario, the rooting of the tree to the oldest HBV EVE (eZHBV_C) suggests the paraphyly of HBV EVEs ( Fig. 4b ) with a potential relationship of eZHBV_M and extant mammalian HBVs that is moderately supported by a bootstrap value of 69% and a Bayesian posterior probability of 0.82. Considering this topology and the apparent absence of HBV EVEs in mammalian genomes, we hypothesize that the common ancestor of Hepadnaviridae probably infected birds and later, following a host switch, one of the hepadnaviral lineages infected mammals. If the assumption of a bird–mammal host switch is correct, Orthohepadnaviridae would constitute a virus taxon that is younger than the Mesozoic eZHBV_C EVE (that is, <94 to <82 MYA) and probably even as young as <12.1 MYA when including the putative phylogenetic position of the Miocene eZHBV_M EVE. 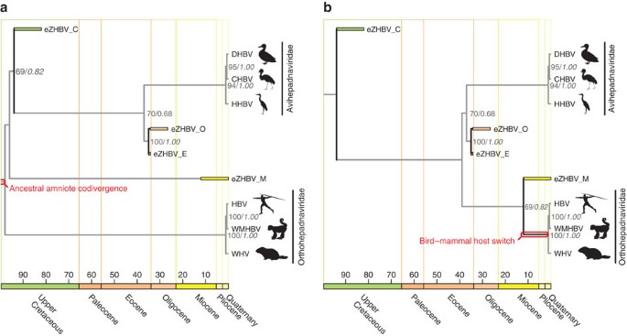Figure 4: Phylogeny of hepatitis B viruses and two scenarios on the origin of mammalian HBVs. (a,b) Consensus tree (grey branches not to scale) of maximum likelihood and Bayesian phylogenetic analyses (Supplementary Fig. S2a,b; for full alignment, seeSupplementary Data 3) of the polymerase protein from extinct eZHBV HASs and extant HBVs. Note that this tree topology is corroborated by our whole-genome nucleotide sequence analysis (Supplementary Fig. S2c). Rooting the tree to mammalian HBVs (a) places the origin of Orthohepadnaviridae before the endogenization of eZHBV_C and implies ancient codivergence of avian and mammalian HBVs. Alternatively, the same tree rooted to the Mesozoic eZHBV_C EVE (b) implies the emergence of Orthohepadnaviridae after a host switch from birds to mammals at some point after the endogenization of eZHBV_C. The representatives of Orthohepadnaviridae are extant HBVs from human (HBV), woolly monkey (WMHBV), and woodchuck (WHV), complemented by representatives of Avihepadnaviridae from duck (DHBV), crane (CHBV) and heron (HHBV). Rectangles are coloured according to the respective geological epoch in the International Stratigraphic Chart and denote the temporal ranges of insertion events. Nodes are labelled with maximum likelihood bootstrap values (in %) and Bayesian posterior probabilities (italicized). Figure 4: Phylogeny of hepatitis B viruses and two scenarios on the origin of mammalian HBVs. ( a , b ) Consensus tree (grey branches not to scale) of maximum likelihood and Bayesian phylogenetic analyses ( Supplementary Fig. S2a,b ; for full alignment, see Supplementary Data 3 ) of the polymerase protein from extinct eZHBV HASs and extant HBVs. Note that this tree topology is corroborated by our whole-genome nucleotide sequence analysis ( Supplementary Fig. S2c ). Rooting the tree to mammalian HBVs ( a ) places the origin of Orthohepadnaviridae before the endogenization of eZHBV_C and implies ancient codivergence of avian and mammalian HBVs. Alternatively, the same tree rooted to the Mesozoic eZHBV_C EVE ( b ) implies the emergence of Orthohepadnaviridae after a host switch from birds to mammals at some point after the endogenization of eZHBV_C. The representatives of Orthohepadnaviridae are extant HBVs from human (HBV), woolly monkey (WMHBV), and woodchuck (WHV), complemented by representatives of Avihepadnaviridae from duck (DHBV), crane (CHBV) and heron (HHBV). Rectangles are coloured according to the respective geological epoch in the International Stratigraphic Chart and denote the temporal ranges of insertion events. Nodes are labelled with maximum likelihood bootstrap values (in %) and Bayesian posterior probabilities (italicized). Full size image Our paleovirological results comprise direct evidence for virus–host coexistence of hepadnaviruses in the Upper Cretaceous, a finding that was so far restricted to bornaviruses and circoviruses (based on shared ancient EVE insertions [2] ), as well as foamy viruses (based on their codivergence with placental mammals [27] ). Above all, this study is the first to present the genome sequence of a Mesozoic paleovirus. Our insights into long-term sequence evolution, genome evolution and hypothetical ancestral hosts change the understanding of the prehistoric evolution of Hepadnaviridae, including the hypothetical origin of mammalian HBVs. We anticipate that this will be of significance to a variety of disciplines involved in studying HBVs or their hosts, including medical research and palaeontology. Additionally, our results emphasize the importance of conducting comprehensive presence/absence analyses in addition to the computational extraction [24] , [25] of paleoviral sequences. With the foreseeable sequencing of a wealth of animal genomes [28] , we expect that our Mesozoic paleovirus genome is just the tip of the iceberg of prehistoric virus genomes. General approach We conducted tBLASTx searches using the DHBV genome (accession code AY494851) as query and the zebra finch genome as database (genomic blast server at the National Center for Biotechnology and Information; http://blast.ncbi.nlm.nih.gov/ ). We complemented these tBLASTx searches by conducting additional searches using the eZHBV fragments of Katzourakis and Gifford [2] and Gilbert and Feschotte [7] as queries. Their eZHBV sequences [2] , [7] had been detected likewise (that is, using tBLASTx searches of DHBV against the zebra finch genome). After we extracted BLAST hits ( E <10 −5 ) including flanking sequences of >5 kb from the taeGut1 assembly in Genome Browser [29] ( http://genome.ucsc.edu/cgi-bin/hgBlat ), we aligned these to the respective orthologous regions of the chicken genome (galGal3 assembly) using MAFFT [30] (FFT-NS-2, version 6, http://mafft.cbrc.jp/alignment/server/index.html ). Based on the insertion sites identified in these sequence alignments, we reconstructed that the total of 16 eZHBV fragments stem from 12 germline infiltration events, as some of these fragments arose via post-insertional duplication of the genomic locus (that is, eZHBVf+g [7] ; eZHBVl+l* [7] ) and others appear to be the result of a big deletion within a beforehand larger eZHBV fragment (that is, eZHBVb+k [7] ; eZHBVi+j [7] ). Eight of these insertion loci exhibited flanking sequences that were suitable for primer design and PCR amplification, that is, well-conserved coding or noncoding regions near the respective eZHBV insertion. Note that we did not consider the previously studied [7] eZHBVj and eZHBVl EVEs, as for these, no absence situation could be amplified [7] , prohibiting the precise dating of these insertions. Subsequent to our comprehensive presence/absence screening of eight eZHBV insertion loci in vitro (see below), we aligned ( Supplementary Data 1 ) all sequences of each orthologous locus using MAFFT (E-INS-i, version 6) and ascertained presence/absence character states ( Supplementary Table S1 ). Our dense taxon sampling (see below) permitted the maximum likelihood-based reconstruction of HASs in MEGA5 [31] (Tamura-Nei model of nucleotide substitution, gamma-distributed rates among sites, five discrete gamma categories, tree topology from Fig. 1 and [13] ) for each orthologous eZHBV insertion shared by more than two species. The resultant ancestral sequences exhibit only a few frameshift mutations and stop codons ( Supplementary Table S2 ). Taxon sampling Our taxon sampling comprises representatives of all major passeroid taxa [32] (including the major ploceid [33] taxa within Passeroidea) on the lineage leading to the zebra finch and thus permits an accurate detection of the upper and lower age boundary of eZHBV endogenization events. For eZHBV_O1-O5 and eZHBV_E, we sampled Anthus gustavi , Carpodacus erythrinus , Prunella modularis (LWL00359), Chloropsis aurifrons , Cinnyris asiaticus and Turdus merula . In the case of eZHBV_M, we additionally sampled Chloebia gouldiae and Ploceus castaneiceps , whereas for eZHBV_C, we included Parus palustris and representatives of the major neoavian lineages [13] , [34] (see Supplementary Table S1 for more information and [13] for species names). Sequence-based verification of species identity was conducted as previously described [13] . In the case of eZHBV_O1, we completed the taxon sampling by using previously published sequences [7] of Chloebia gouldiae , Junco hyemalis and Cyanomitra olivaceus from GenBank ( http://www.ncbi.nlm.nih.gov/Genbank/ ; accession codes HQ116567 , HQ116565 , and HQ116564 ). In vitro screening We conducted a comprehensive in vitro screening for our eight eZHBV insertion loci that is consistent with the procedures described by Suh et al. [13] in their study of retroposon presence/absence patterns. Briefly, eZHBV insertion loci were amplified via touchdown PCR, followed by purification and cloning of the PCR amplicons, and subsequent sequencing of the cloned fragments [13] . In the case of the large eZHBV_C insertion locus, a modified touchdown PCR protocol was used (5 min elongation time instead of the 80 s in the normal touchdown PCR protocol [13] ), as well as various primers ( Supplementary Table S4 ) for amplification and/or direct sequencing of the resultant PCR amplicons. Sequence analyses Owing to the large size of many eZHBV_C PCR amplicons (3.6–4.3 kb), we sequenced the full eZHBV_C locus sequence in four distantly related [13] , [34] neoavians (that is, Nestor notabilis , Buteo lagopus , Larus ridibundus and Columba palumbus ) and used these sequences for HAS reconstruction of eZHBV_C. The other complete neoavian sequences (that is, Taeniopygia guttata , Cinnyris asiaticus , Alcedo atthis , Apus apus and Chrysolampis mosquitus ) were not included due to the presence of large tandem duplications or large secondary deletions within the HBV-derived sequence. We calculated pairwise distances of eZHBV HASs using MEGA5 (maximum composite likelihood, inclusion of transitions + transversions, uniform rates among sites, homogeneous patterns among lineages, complete deletion of alignment gaps). Dividing these by the mean time interval between the endogenization of the respective older and younger paleovirus, we estimated nucleotide substitution rates of the different prehistoric chapters of HBV evolution ( Supplementary Table S3 ). For further in-depth sequence analyses, amino-acid sequences of eZHBV paleoviruses were estimated after removal of frameshifts (that is, exclusion of frameshifting insertions, insertion of alignment gaps in frameshifting deletions) and internal stop codons (that is, replacement by ‘X’). Sequence conservation graphs were compiled on the basis of amino-acid sequence alignments of pol, preS/S, preC/C ORFs ( Supplementary Data 2 ) and by plotting extant HBV sequences (DHBV, CHBV, HHBV, HBV, WMHBV, WHV) to the Mesozoic eZHBV_C paleovirus. We coded sequence identities with the value ‘1’, whereas non-identical alignment positions (including gaps) received a value of ‘0’. Perfect (that is, 100%) conservation of an alignment position thus corresponds to a cumulative value of ‘6’. Note that alignment gaps in the reference sequence (eZHBV_C) were treated as missing data and therefore marked with grey background in Fig. 3 (panels b–d). Finally, we performed phylogenetic sequence analyses of the pol protein of HBV EVEs and extant HBVs, as all but one (eZHBV_O1) of the eZHBV EVEs map to at least a part of this hepadnaviral ORF. To obviate problems arising from too short sequences of the four Oligocene EVEs overlapping with the pol ORF (eZHBV_O2-O5), we concatenated these into a chimaeric sequence, as we assume that these EVEs are likely to be closely related and of similar age. We compiled an alignment of complete and partial pol protein sequences ( Supplementary Data 3 ) using MAFFT (E-INS-i, version 6) alignment and manual rechecking. Following model testing in MEGA5 that revealed WAG as most and JTT as second-most appropriate model, various phylogenetic analyses were performed using the CIPRES Science Gateway [35] ( http://www.phylo.org/portal2/ ) and TOPALi [36] (version 2.5). Irrespective of the model used (WAG or JTT), maximum likelihood (RAxML [37] ) and Bayesian (MrBayes [38] ) inferences of phylogeny constantly yielded the same topology (two examples are shown in Supplementary Fig. S2a,b ). To evaluate the putative distant relationship of the youngest paleovirus (eZHBV_M) and the other eZHBV EVEs, we furthermore conducted a Bayesian sequence analysis (with GTR as best-fit model) of aligned nucleotides of whole-genome sequences (extant HBVs and eZHBV_C) plus eZHBV genome fragments. The resultant tree ( Supplementary Fig. S2c ) exhibits the same tree topology, except for a basal polytomy involving eZHBV_M. Thus, eZHBV_M forms a distinct hepadnaviral lineage that, if it is indeed related to mammalian HBVs, implies a relatively recent bird–mammal host switch. How to cite this article: Suh, A. et al. The genome of a Mesozoic paleovirus reveals the evolution of hepatitis B viruses. Nat. Commun . 4:1791 doi: 10.1038/ncomms2798 (2013).